Elucidating the genomic architecture of AsianEGFR-mutant lung adenocarcinoma through multi-region exome sequencing EGFR -mutant lung adenocarcinomas (LUAD) display diverse clinical trajectories and are characterized by rapid but short-lived responses to EGFR tyrosine kinase inhibitors (TKIs). Through sequencing of 79 spatially distinct regions from 16 early stage tumors, we show that despite low mutation burdens, EGFR -mutant Asian LUADs unexpectedly exhibit a complex genomic landscape with frequent and early whole-genome doubling, aneuploidy, and high clonal diversity. Multiple truncal alterations, including TP53 mutations and loss of CDKN2A and RB1 , converge on cell cycle dysregulation, with late sector-specific high-amplitude amplifications and deletions that potentially beget drug resistant clones. We highlight the association between genomic architecture and clinical phenotypes, such as co-occurring truncal drivers and primary TKI resistance. Through comparative analysis with published smoking-related LUAD, we postulate that the high intra-tumor heterogeneity observed in Asian EGFR -mutant LUAD may be contributed by an early dominant driver, genomic instability, and low background mutation rates. Although comprehensive genomic sequencing studies have identified recurrent somatic alterations in LUAD [1] , [2] , [3] , [4] , [5] , [6] , [7] , [8] , majority has been based on single-tissue samples and lack the resolution to evaluate clonal architecture. Further, certain clinical phenotypes, such as never-smoker Asian EGFR -mutant LUAD are under-represented in these cohorts [1] , [2] , [3] , [4] , [5] , [6] , [7] , [8] . Activating mutations in the epidermal growth factor receptor ( EGFR ) are the most common therapeutically tractable driver mutation in lung adenocarcinomas (LUAD) with distinct ethnic differences, occurring at higher frequencies in Asians (40–60%) compared to Caucasians (7–10%) [9] , [10] , [11] , [12] . Due to the preponderance of never smokers, EGFR -mutant LUADs are often associated with low-mutation burdens. On the contrary, the copy number landscape has been shown to harbor considerable genomic complexity [13] , [14] , [15] , although the extent to which these observations are confounded by intra-tumor heterogeneity (ITH) is unclear. While it is feasible to computationally resolve clonal composition in single-tissue samples [16] , [17] , [18] , these methods lack sensitivity and specificity especially in tumors with high ITH, where regionally dominant clones may exist. More recently, multi-region sequencing studies on smoker dominated Caucasian non-small cell lung cancers (NSCLC) have revealed high-mutation burden and low ITH [19] , [20] , [21] —primarily attributed to inordinately long trunks (representing mutations shared by all regions of a tumor) as a result of accruing multiple passenger and driver alterations from chronic tobacco exposure. On the other hand, late diversification was contributed by branch/private driver alterations (mutations present in few but not all regions of tumor/present in single region of tumor) and increased APOBEC activity, representing evolutionary processes that are potentially amenable to therapeutic targeting [16] , [19] . The extent of ITH, and the factors that drive cancer evolution, is of clinical interest as it has been inextricably linked to treatment failure [22] , [23] . In EGFR -mutant LUAD, selection pressures imposed by targeted therapies can either result in expansion of pre-existing rare TKI resistant subclones (e.g., cells harboring EGFR T790M or MET amplifications) or be acquired stochastically [24] , [25] , [26] . The rapid emergence of resistance to EGFR TKIs [27] , [28] seems counter intuitive in the context of low-mutation burden, and the impact of intra-tumor heterogeneity on the extent of tumor shrinkage and eventual emergence of drug resistance is not well established. Here we present the first comprehensive description of the genomic architecture of EGFR -mutant LUAD through multi-region exome sequencing and SNP arrays on 16 tumors. Despite low-mutation burdens in these predominantly never-smoker oncogene-driven LUADs, we demonstrate an under-appreciated level of genomic complexity, both in terms of copy number landscape, as well as relatively high-proportional ITH due to early diversification in these tumors. Through integrative genomics, we show that early EGFR and TP53 mutations are often followed by genome doubling events, with ongoing genomic instability typified by a variegated copy number landscape and late high-amplitude amplifications and deletions. We further highlight how multiple co-occurring drivers may portend poor clinical outcomes, including primary EGFR TKI resistance. By comparing the clonal architecture of our EGFR -mutant LUAD with that of previously published smoking-related LUAD, we provide insights into determinants of ITH and suggest that the evolutionary trajectories of LUADs are shaped by cumulative effects of background mutation rates, strength and timing of driver mutations and ongoing genomic instability. Spatio-temporal relationship of mutations relative to EGFR We subjected 16 surgically resected stage I–II treatment naive EGFR -mutation positive Asian LUAD cases (15 never smokers) to multi-sector whole-exome sequencing. A total of 79 sectors with 3–11 regions from each tumor were sequenced (mean depth 114X; Supplementary Fig. 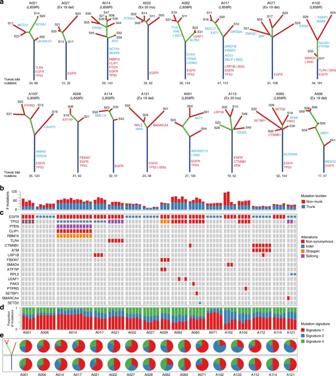Fig. 1 Landscape of clonal and subclonal mutations in AsianEGFR-mutant tumors.aPhylogenetic trees generated for the 16 AsianEGFR-mutant LUADs. Trunks, branches and tips are depicted in blue, green, and red, respectively, while non-silent mutations carrying LUAD specific drivers are in red and other cancer drivers are in blue (Methods section). All patients are never-smokers except A103 (marked *) who was a light ex-smoker. Truncal mutation burden followed by total mutation burden for all sectors is indicated below the trees.bBar plot representing truncal and non-truncal mutation burden per sector.cOncoprint heatmap for mutations in LUAD drivers depicting the presence (see color legend) or absence (gray box) and type of non-silent mutation.dProportions of the three mutation signatures identified for each sector. Signature numbers are according to the COSMIC nomenclature.ePie charts representing contribution of the three mutation signatures in early (trunk) and late (branch/private) mutations 1 ; Supplementary Table 1 ). Somatic single-nucleotide variants (SNVs) and indels were identified and subjected to target deep sequencing (mean depth of 3860X). In all, 1450 SNVs and 71 indels were confirmed, affecting exons of 1318 genes (Supplementary Data 1 ), from which phylogenetic trees and mutation heatmaps were generated (Fig. 1a, b ; Supplementary Fig. 2 ). Fig. 1 Landscape of clonal and subclonal mutations in Asian EGFR -mutant tumors. a Phylogenetic trees generated for the 16 Asian EGFR -mutant LUADs. Trunks, branches and tips are depicted in blue, green, and red, respectively, while non-silent mutations carrying LUAD specific drivers are in red and other cancer drivers are in blue (Methods section). All patients are never-smokers except A103 (marked *) who was a light ex-smoker. Truncal mutation burden followed by total mutation burden for all sectors is indicated below the trees. b Bar plot representing truncal and non-truncal mutation burden per sector. c Oncoprint heatmap for mutations in LUAD drivers depicting the presence (see color legend) or absence (gray box) and type of non-silent mutation. d Proportions of the three mutation signatures identified for each sector. Signature numbers are according to the COSMIC nomenclature. e Pie charts representing contribution of the three mutation signatures in early (trunk) and late (branch/private) mutations Full size image EGFR mutations were confirmed to be truncal events (mutations present in all sectors of a tumor) in every case regardless of the mutation type (L858R, exon 19 deletion or exon 20 insertion), underscoring its role as an early tumor initiating driver event (Fig. 1a , Supplementary Data 2 ). Besides EGFR , TP53 was the most recurrently mutated gene with mutations in 9 out of 16 tumors, of which eight were truncal events (Fig. 1a, c ; Supplementary Data 1 , 2 ). Only 17 other LUAD-specific driver genes (those found to be recurrently mutated in LUAD; Methods section) were found mutated, of which 7 (<50%) featured as truncal events in 4/16 tumors (Fig. 1c ). Further, just two of these 17 driver genes ( LRP1B and CTNNB1 ) were recurrently mutated across two patients (Fig. 1a, c , Supplementary Data 1 , 2 ). Interestingly, both CTNNB1 mutations (S37C and K335I, Supplementary Data 1 ) are known to be oncogenic and deregulate beta-catenin activity [29] , [30] possibly contributing to EGFR -mediated tumorigenesis [31] . In addition, we find infrequent mutations that have recently been shown to have functional roles. For example, the private mutation affecting D323 residue of AKT1 (found in A001, Fig. 1a , Supplementary Data 2 ) has been shown to be activating/oncogenic [32] contributing to erlotinib resistance in EGFR -mutant PC-9 cells [33] . Loss-of-function of MED12 has been implicated in resistance to EGFR TKIs [34] suggesting that the truncal MED12 frameshift deletions in A006 and the private MED12 mis-sense mutation (predicted to be damaging; Supplementary Data 1 , 2 ) in A021 might be candidates for resistance inducing mutations. However, we did not find any common resistance mutations like the T790M in EGFR , in any sector, likely due to their rare occurrence in treatment naive samples that are beyond the detection limits of our sequencing parameters [24] . Multi-region sequencing reveals high ITH in EGFR -mutant LUAD Using the percentage of branch/private mutations—a common measurement of ITH [19] , [20] , [35] (we term this proportional ITH or pITH), we found a median of 62.3% heterogeneity (range: 32.26–82.2%) in our largely never-smoker Asian EGFR -mutant LUADs, contrary to previous findings of low ITH in LUAD (~30% branch mutations; Fig. 1a, b , Supplementary Fig. 2 , Supplementary Data 2 ) [19] , [20] . To eliminate any biases arising from different analysis pipelines, we re-analysed the data from the two earlier reports using our pipelines (Supplementary Fig. 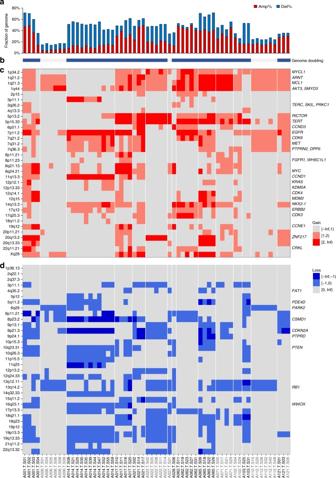Fig. 2 Genomic instability and variegated copy number landscape ofEGFR-mutant tumors.aBar plot representing the fraction of genome altered by copy number alterations relative to ploidy of the sector, which is termed as the genomic instability index (GII).bBar showing genome doubling status. Blue indicates significant evidence for genome doubling (Supplementary Data3, Methods section) and gray indicates no genome doubling.cHeatmap depicting gains in known driver or recurrently amplified cytobands in LUAD (Methods section). Light red represents gain in one copy beyond the ploidy while dark red represents gain in ≥2 copies beyond the ploidy.dHeatmap depicting losses in known driver or recurrently amplified cytobands in LUAD (Methods section). Light blue represents loss of one copy relative to the ploidy while dark blue represents loss of ≥2 copies beyond the ploidy. Samples for all panels are as depicted ind.TP53wild-type samples are depicted in gray 3 , Supplementary Table 2 ) and confirmed the differences in pITH even after controlling for the number of sectors per tumor (Supplementary Fig. 4 ). Consistent with the higher pITH, we found an average increase of 37% in mutation burden upon sequencing three random sectors in EGFR mutation positive Asian LUAD compared to only 17% increase in smoker dominated Caucasian LUAD (Supplementary Fig. 5 ), underscoring the higher relative burden of branch/private mutations in the former. APOBEC activity is infrequently observed in EGFR -mutant LUAD We next examined the mutational signatures associated with early and late genetic events in Asian EGFR- mutant LUAD. Among the three mutation signatures identified in our patients (Supplementary Fig. 6 ) the age-associated molecular clock like signature-1 [36] , [37] dominated the mutational landscape of these 16 EGFR -mutant patients including the light ex-smoker A103 (Fig. 1d ). The distribution of signatures between early (trunk) and late events (branch/private) was heterogeneous across patients (Fig. 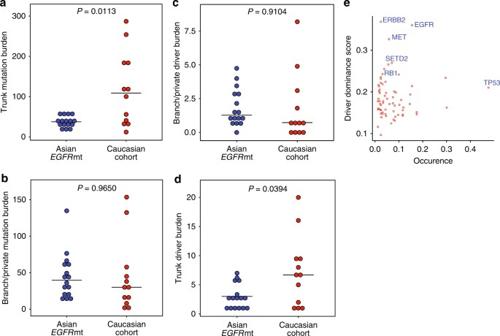Fig. 3 EGFRis a dominant driver with few co-drivers. Dot plots comparing mutation burden onatrunk andbbranches between the AsianEGFR-mutant and smoker dominated Caucasian cohorts19,20.cDot plot comparing number of branch/private mutated drivers (extended driver list) between the EGFR-mutant and smoker dominated Caucasian cohorts19,20. Welch’st-test was used to compare the two groups.dDot plot showing thatEGFR-mutant LUADs have significantly fewer truncal drivers (extended driver list; Welch’st-test) compared to smoker Caucasian LUADs. Three random sectors were picked 20 times iteratively and averages of the iterations are represented as circles ina–d. Horizontal line indicates the median for that cohort.e“Driver dominance score” measuring driver self-sufficiency for each of 78 LUAD driver genes calculated across published 412 tumors3,4is plotted against the fraction of patients carrying the mutated driver 1e ) and collectively we did not find significant change for any signature between the early and late events (signature-1: P = 0.43; signature-2: P = 0.62; signature-4: P = 0.08, paired t -test). However, 4 of 16 patients (A102, A103, A114, and A121) demonstrated relatively higher contribution of APOBEC activity (signature-2) in late subclonal events (Fig. 1e ). Of note, marked spatial heterogeneity was observed in one patient (A102)—a TP53 wild-type non-smoker, where two out of four sectors showed considerably increased contribution of APOBEC signature and disproportionately higher sector-specific mutational burden (Fig. 1b, d, e ). These observations support the role of increased activity of APOBEC family of enzymes as a putative mechanism driving subclonal diversification [16] , [19] , [20] , although only in a minority of EGFR -mutant cases. EGFR -mutant LUAD display a variegated copy number landscape We successfully profiled somatic copy number alterations (SCNA) for 61 of the 79 tumor sectors across 15 patients (Fig. 2 , Supplementary Fig. 7 ). Using a genome instability index (GII, defined as fraction of the genome altered by SCNAs, copy change ≥1 relative to ploidy; see Methods section), we found that majority of tumors showed moderate to high-genomic instability (median of 48.1% per tumor sector, Fig. 2a ), as well as frequent whole-genome doubling (WGD) events (12 of 15 tumors, except A006, A027, and A112; Fig. 2b , Supplementary Data 3 ). Interestingly, we find WGD to be a truncal event (Fig. 2b , Supplementary Data 3 ) wherever present, suggesting them to occur early in tumorigenesis, consistent with its implications as a common route leading to genomic and chromosomal instability (CIN), fueling intra-tumor heterogeneity [6] , [38] , [39] . Using the eleven tumors with SCNA data in at least three sectors, we observed 40.5% of cytobands and 41.35% of genes to be affected by late branch or private copy number alterations (Supplementary Fig. 8 ; Supplementary Data 4 , 5 ; Methods section). While we saw little variance in GII scores across sectors (Fig. 2a ), majority of the SCNAs contributing were low-copy gains and losses (copy change = 1 relative to ploidy; Supplementary Figs 7 , 9 ). In contrast, while a median of only 7.2% of genome was affected by high-copy gains and losses (copy change ≥2 relative to ploidy; defined as adGII or amplification and deletion based genomic instability index; Supplementary Fig. 9 ), we observed a significantly higher variance in adGII scores across sectors of a tumor compared to GII scores ( P = 5 × 10 −4 , Welch’s t -test; Supplementary Fig. 10 ) suggesting continuous evolution of copy number landscape with late increase in amplitude of the alterations. Focusing on genes where amplifications have been reported as putative resistance mechanisms to EGFR TKIs [25] , [40] , we find low-copy gains for MET , ERBB2 , and HGF genes in 12/15 patients (Supplementary Fig. 11 ). While some were truncal events, five patients displayed ≥5 copies in either of these three genes in at least one sector confirming that these amplifications do pre-exist subclonally in some tumors (Supplementary Fig. 11 , Supplementary Data 4 ), and may contribute to a drug tolerant state. Fig. 2 Genomic instability and variegated copy number landscape of EGFR -mutant tumors. a Bar plot representing the fraction of genome altered by copy number alterations relative to ploidy of the sector, which is termed as the genomic instability index (GII). b Bar showing genome doubling status. Blue indicates significant evidence for genome doubling (Supplementary Data 3 , Methods section) and gray indicates no genome doubling. c Heatmap depicting gains in known driver or recurrently amplified cytobands in LUAD (Methods section). Light red represents gain in one copy beyond the ploidy while dark red represents gain in ≥2 copies beyond the ploidy. d Heatmap depicting losses in known driver or recurrently amplified cytobands in LUAD (Methods section). Light blue represents loss of one copy relative to the ploidy while dark blue represents loss of ≥2 copies beyond the ploidy. Samples for all panels are as depicted in d . TP53 wild-type samples are depicted in gray Full size image We next estimated the timing of recurrent truncal mutations relative to WGD and copy number alterations using a published algorithm [16] . The inferred cancer cell fractions and mutant allele copy numbers suggest that EGFR and TP53 mutations occurred prior to WGD and local SCNA (Supplementary Data 6 ), underscoring the founding role of these two drivers during tumorigenesis. Notably, in the nine tumors harboring mutations in TP53 , all had undergone WGD (compared to 3 out of 6 in TP53 wild type (wt)) (Fig. 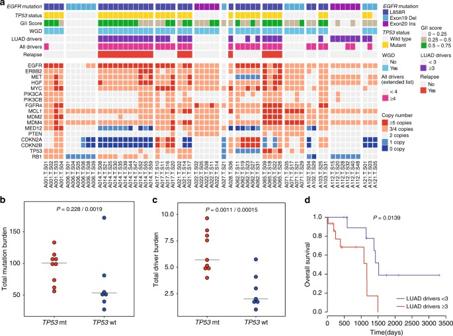Fig. 4 TP53mutations, genomic instability, high-driver burden lead to poor outcome.aLower panel is a heatmap representing number of copies for selected genes involved in EGFR TKI resistance or associated with prognosis. Upper panel represents features of a tumor which are associated with patient outcome likeTP53mutation status, genomic instability index, presence of whole-genome doubling, above and below median number of drivers (LUAD specific or extended driver list) and the relapse status. All these features tend to coincide in many tumors.bTotal mutation burdens andcdriver burdens (extended driver list) are compared betweenTP53mutant (mt) and wild-type (wt) tumors. Three random sectors were picked iteratively (n= 20) and averages across iterations are represented inbandc. The firstp-value is taking all 16 patients into consideration and the secondp-value is after eliminating the outlier A102 in the analysis.P-values are calculated using Welch’st-test.dSurvival plots using TCGA LUADEGFR-mutant cases (those with non-silent mutations in tyrosine kinase domain,n= 26)4after stratifying above or below median number of LUAD drivers (median = 3).P-value fromχ2-test is indicated 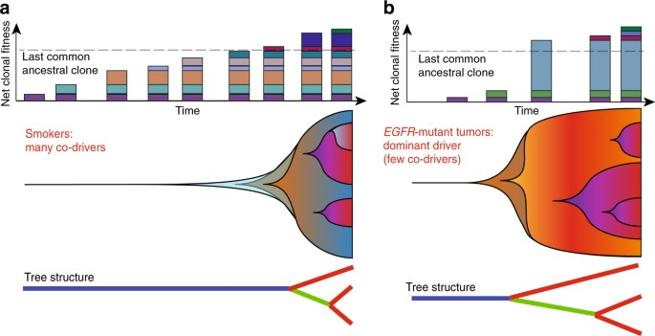Fig. 5 Schematic of evolutionary trajectories in smokers andEGFR-mutant non-smoker tumors.aIn smokers, accumulation of many truncal mutations and drivers before branched evolution. Top: driver mutations are represented as colored rectangles. The dashed line indicates the point of diversification on the tree or the last common ancestral clone (carrying the last truncal driver mutation). Middle: shaded background represents clonal expansion (y-axis) as mutations accumulate (x-axis) in individual clones (colors). Bottom: schematic representation of phylogenetic mutation tree.bThe non-smoker scenario where a dominant driver likeEGFRis hit early leading to a big fitness advantage, fewer clonal sweeps and early diversification. Panel structure as ina. In both scenarios, evolutionary trajectory is influenced by clonal dynamics, which in turn is related to competitive fitness of the individual cell populations. Example of such factors include but are not limited to mutations rates, driver nature, cytokine milieu, immune cell infiltration, and metabolic conditions 2b , Supplementary Data 3 ) and were further associated with significantly higher genomic instability ( P = 0.0131, Welch’s t -test; Supplementary Fig. 12 , Fig. 2a ). Overall, our data reveal how EGFR -mutant LUAD can harbor a complex copy number landscape that can be influenced by TP53 mutation status—and undergoes continuous evolution over time with early low-copy gains and losses followed by late high-amplitude changes. Early SCNA converge on disruption of cell cycle control We next examined the recurrent copy number changes, focusing on the cytobands with recurrent SCNAs and driver cytobands identified in previous large scale studies [4] , [6] , [7] , [8] , [41] . We found gains in multiple cytobands from chromosome 1, 5p, and 7p containing important driver genes like TERT , EGFR , anti-apoptotic MCL1 and TP53 inactivator MDM4 as the most recurring truncal events in more than half of the tumors evaluated for SCNA ITH (Fig. 2c ; Supplementary Fig. 7 ; Supplementary Data 4 , 5 ). Truncal deletion events were observed in regions, such as 13q14.2, 9p21.3 and 10q23.31 containing known tumor suppressors like RB1 , CDKN2A , and PTEN (Fig. 2d ). Among these, 9p21.3 containing CDKN2A/2B carried truncal losses relative to ploidy across six tumors and was the only known driver region with truncal homozygous deletions in two tumors (Fig. 2d ; Supplementary Fig. 13a ; Supplementary Data 4 , 5 ). Interestingly, all TP53 wild-type tumors had truncal losses affecting the 13q14.2 region containing RB1 (Fig. 2d ) and four of these tumors had loss of heterozygosity (LOH) containing just single copy of this gene (Supplementary Fig. 13b ). In addition to recurrent somatic mutations in TP53 , we further observed recurrent truncal LOH in 7/11 tumors including those without any mutations (Supplementary Fig. 13c ). In EGFR -mutant tumors with TP53 mutations, 6/9 tumors were found to have LOH and loss in copy number in RB1 region (3 tumors with potentially truncal LOH; Supplementary Fig. 13b ). Overall these findings implicate disruption of the RB1/CDKN2A/TP53 control axis of the cell cycle G1/S and apoptosis checkpoints as an early tumor initiating event in EGFR -mutant LUADs. Determinants of high ITH in EGFR mutant LUAD Although lower pITH in the smoker enriched Caucasian cohort (Supplementary Fig. 4 ) can be explained by the higher number of smoking induced truncal mutations during the life history of a tumor (Fig. 3a ), the comparable absolute mutation burden on the branches between smoker Caucasian and our non-smoker cohorts (Fig. 3b ) was unexpected. Given that smoking related tumors can harbor up to 10 times the mutation burden of non-smoking counterparts [2] , [3] , the comparable level of genetic diversity (number of branch mutations) attained by EGFR -mutant LUAD was quite striking. In exploring potential reasons for the unexpectedly high-branch mutations in EGFR -mutant LUAD, we did not find enrichment for subclonal drivers (Fig. 3c ) nor consistent increase in APOBEC-associated mutagenesis, the latter found in only a subset of tumors (Fig. 1d, e ). Fig. 3 EGFR is a dominant driver with few co-drivers. Dot plots comparing mutation burden on a trunk and b branches between the Asian EGFR -mutant and smoker dominated Caucasian cohorts [19] , [20] . c Dot plot comparing number of branch/private mutated drivers (extended driver list) between the EGFR-mutant and smoker dominated Caucasian cohorts [19] , [20] . Welch’s t -test was used to compare the two groups. d Dot plot showing that EGFR -mutant LUADs have significantly fewer truncal drivers (extended driver list; Welch’s t -test) compared to smoker Caucasian LUADs. Three random sectors were picked 20 times iteratively and averages of the iterations are represented as circles in a – d . Horizontal line indicates the median for that cohort. e “Driver dominance score” measuring driver self-sufficiency for each of 78 LUAD driver genes calculated across published 412 tumors [3] , [4] is plotted against the fraction of patients carrying the mutated driver Full size image Based on the fewer truncal drivers observed in EGFR -mutant LUAD compared to smoker dominated Caucasian LUAD (Fig. 3d ), we surmised that EGFR mutations may require fewer co-drivers for clonal expansion. To test whether EGFR tends to be dominant (i.e., ‘self-sufficient’) and has less co-drivers across tumors compared to other LUAD drivers, we developed a “driver dominance score”, which measures the number of co-occurring drivers for each defined driver gene per tumor. Drivers with higher dominance score will tend to have less co-drivers across cases (Methods section). Applying this procedure across 412 published LUADs [3] , [4] , EGFR ranked second, underscoring its role as a dominant (genetically self-sufficient) LUAD driver (Fig. 3e ). We next explored the relevance of this score to clear cell renal cell carcinoma (ccRCC), a tumor that similarly has a recurrent truncal alteration (VHL), comparable mutation burdens, and early diversification (high pITH 67.95%) [35] . In agreement with our hypothesis, VHL too ranked as the most dominant driver in ccRCC (Supplementary Fig. 14 ), when we applied the same “driver dominance” metric to exome-wide mutation data from the TCGA ccRCC cohort [42] . These data raise the possibility that early dominant tumor-initiating events can contribute at least in part, to shaping the distinct genomic architecture of tumors. Taken together, our findings from multi-region sequencing of EGFR -mutant LUAD suggest that a dominant truncal driver, in the context of low-mutation rates and high-genomic instability, likely results in early clonal selection with subsequent high-intra-tumor heterogeneity. Impact of genomic architecture on clinical trajectories Out of the five patients who relapsed during the course of this study after surgery (Supplementary Table 1 ), four carried truncal mutations in TP53 (A021, A028—both Stage IA; A014—Stage IB; A065—Stage IIA), consistent with its previously reported association with poor outcomes [10] , [43] , [44] . The remaining patient who relapsed (A114) had stage IIB disease and prognostically unfavorable clinical features, including lymphovascular invasion, involvement of hilar and intrapulmonary lymph nodes, and was the largest tumor in our series at 6.0 cm (Supplementary Table 1 ). In addition to the previously described association with WGD and GII (Fig. 2a, b , Supplementary Fig. 12 , Fig. 4a , top panel), we found that TP53 , EGFR double-mutant LUAD also harbored higher mutation and driver burdens, both on the trunk and branches (Fig. 4a , top panel, Fig. 4b, c, Supplementary Fig. 15 ), where out of 9 tumors with ≥3 LUAD specific driver mutations, 8 were TP53 -mutant. Majority of these drivers were truncal (70.5%, 31/44) although some patients had disproportionately more branch/private mutations, such as patient A121 who harbored a branch TP53 mutation, and A065 who carried four different LUAD driver mutations in four different sectors (Fig. 1a, c , Supplementary Data 7 ). Fig. 4 TP53 mutations, genomic instability, high-driver burden lead to poor outcome. a Lower panel is a heatmap representing number of copies for selected genes involved in EGFR TKI resistance or associated with prognosis. Upper panel represents features of a tumor which are associated with patient outcome like TP53 mutation status, genomic instability index, presence of whole-genome doubling, above and below median number of drivers (LUAD specific or extended driver list) and the relapse status. All these features tend to coincide in many tumors. b Total mutation burdens and c driver burdens (extended driver list) are compared between TP53 mutant (mt) and wild-type (wt) tumors. Three random sectors were picked iteratively ( n = 20) and averages across iterations are represented in b and c . The first p -value is taking all 16 patients into consideration and the second p -value is after eliminating the outlier A102 in the analysis. P -values are calculated using Welch’s t -test. d Survival plots using TCGA LUAD EGFR -mutant cases (those with non-silent mutations in tyrosine kinase domain, n = 26) [4] after stratifying above or below median number of LUAD drivers (median = 3). P -value from χ 2 -test is indicated Full size image Interestingly, patient A014, who in addition to a TP53 mutation, carried the highest number of truncal LUAD drivers (five drivers, Fig. 1a, c ) and displayed the worst clinical outcome in our series, relapsing in just 4 months. Upon subsequent treatment with gefitinib after relapse, only minor tumor shrinkage was elicited in this patient, with ensuing disease progression and demise within 5 months, consistent with primary TKI resistance. A patient-derived cell line (named 471L cells) from the initial resected primary tumor, was confirmed to harbor the same truncal alterations through targeted re-sequencing (Supplementary Data 8 ) and similarly exhibited gefitinib resistance (IC 50 9.79 µM, as compared to the TKI-sensitive PC-9 cell line, IC 50 0.001 µM, Supplementary Fig. 16 ). Thus, through the clinical course of the patient and patient-derived cell line, we provide functional evidence for the potential role of multiple truncal co-drivers in primary resistance. To validate the impact of number of driver mutations and mutation burdens on outcome, we next examined EGFR -mutant patients from the published TCGA cohort [4] . Stratifying patients with respect to number of either driver or all mutations, demonstrated shorter overall survival for cases with higher number of drivers (Fig. 4d ; P = 0.0139, χ 2 -test) or higher overall mutation burdens (Supplementary Fig. 17 ; P = 0.0493, χ 2 -test). Taken together, our data suggest that in EGFR -mutant LUAD, an early TP53 mutation may impact clinical outcomes through facilitating genomic instability and the acquisition of additional co-occurring driver events. On the opposite end of the clinical spectrum, of the seven patients with TP53 wt tumors, five harbored only the activating EGFR mutation as the single-truncal driver. One of these patients, A006 charted an indolent clinical course, having been radiologically diagnosed with ground glass opacities for 5 years prior to surgery. Here, the genomic landscape was distinctly “silent”, with the lowest GII score, no WGD, low-mutation burden and no LUAD co-drivers (Figs. 1 a–c, 2a, b , 4a , Supplementary Data 2 , 3 ). Despite the limited cohort size, these findings illustrate how a spectrum of clinical trajectories might be dictated by the course of genomic events and traits, including TP53 mutations, presence of multiple truncal drivers, aneuploidy, and associated genomic instability. Through multi-region sequencing, we have, for the first time, characterized the clonal and subclonal genomic landscape of Asian EGFR mutation positive LUAD. Despite the low somatic mutation burden, EGFR -mutant LUADs exhibit a heterogeneous genomic landscape characterized by (i) high proportion of late branch and private mutations and (ii) large proportion of genome altered through a combination of early genome doubling events and low-copy gains and losses, followed by late sector-specific copy number changes. Our findings illustrate how timing of genomic events and mutation rates can influence the natural history and diverse clinical trajectories of EGFR -mutant LUAD. Founding mutations in EGFR and frequent early TP53 mutations coupled with other truncal alterations deregulating the cell cycle and evading cell death, facilitate tolerance of pervasive WGD and CIN. Despite a relatively high fraction of branch mutations in these treatment naïve tumors, we generally observed a low prevalence of subclonal drivers or putative resistance mutations (e.g., D323N in AKT1), consistent with a neutral evolution model [45] . While the truncal activating mutations in EGFR provide high-response rates to the targeted EGFR TKIs, these responses are often short-lived [27] , [28] unlike those to Imatinib in BCR-ABL1 fusion driven chronic myeloid leukemia (CML) [46] , [47] . Although the determinants of durability of response in CML remain poorly understood, current studies suggest that the burden of point mutations and SCNAs is moderate in CML compared to solid tumors [48] which possibly contributes to the longer TKI responses of CML compared to LUAD patients [47] . As a result of ongoing genomic instability in EGFR -mutant LUAD, we observed late sector specific copy number amplifications in previously reported genes mediating TKI resistance such as ERBB2 , MET , and HGF [25] , [40] , providing a potential substrate for developing a drug tolerant state. In addition, the subclonal nature of high-amplitude amplifications and deletions underscores the challenge in interpreting gene copy number thresholds e.g., MET and ERBB2 , from single biopsies in NSCLC [49] . Importantly, we implicate the role of multiple co-truncal drivers in a patient exhibiting primary EGFR TKI resistance, with validation in a corresponding patient-derived cell line, and by supporting findings from public data sets. It is thus plausible that co-existing truncal drivers may be associated with a propensity for primary resistance, while minor clones with additional drivers or resistance-mediating alterations can emerge later after initial tumor response to EGFR TKIs. However, larger sample sizes with more functional validations will be needed to test this and to decouple the effects of different genomic features like TP53 mutations, driver burdens and GII. An unexpected observation was the high pITH in never-smoker-enriched EGFR -mutant LUAD with comparable branch/private mutation burden to smoker LUADs. Although our study does not allow delineation of all the intermediate steps and selective sweeps preceding the final clonal composition, it nevertheless illustrates the contrasting life histories and a distinct evolutionary trajectory of EGFR -mutant LUAD, compared to smoking-related LUADs [19] , [20] . In the smoking scenario, a tumor-initiating cell population acquires mutations at a high rate and hence accumulates a large number of passenger and relatively weak driver mutations, with low likelihood for early acquisition of dominant drivers like EGFR (Fig. 5a ). On the background of high-mutation rates, it is possible that, consecutive drivers are gained within a time frame that results in selective clonal sweeps with eventual population expansion and long trunks as previously observed (Fig. 5a ). In contrast, in an oncogene-driven never-smoker LUAD, a dominant driver e.g., EGFR mutation, in the context of low-mutation rates—is sufficient to allow expansion of early tumor cells with few co-drivers. As a result of low-mutation rates, subsequent drivers occur late and are less likely to cause complete sweeps, resulting in shorter trunks and early diversification (Fig. 5b ). Given the inter-patient differences in genomic architecture in our current series, further studies are required to unravel the additional determinants of clonal dynamics for each patient, such as the cytokine milieu [50] , immune cell infiltration [51] and differential metabolic phenotypes in the tumor microenvironment [52] ; as well as how these may relate to selective pressures imposed by anticancer therapies. Fig. 5 Schematic of evolutionary trajectories in smokers and EGFR -mutant non-smoker tumors. a In smokers, accumulation of many truncal mutations and drivers before branched evolution. Top: driver mutations are represented as colored rectangles. The dashed line indicates the point of diversification on the tree or the last common ancestral clone (carrying the last truncal driver mutation). Middle: shaded background represents clonal expansion ( y -axis) as mutations accumulate ( x -axis) in individual clones (colors). Bottom: schematic representation of phylogenetic mutation tree. b The non-smoker scenario where a dominant driver like EGFR is hit early leading to a big fitness advantage, fewer clonal sweeps and early diversification. Panel structure as in a . In both scenarios, evolutionary trajectory is influenced by clonal dynamics, which in turn is related to competitive fitness of the individual cell populations. Example of such factors include but are not limited to mutations rates, driver nature, cytokine milieu, immune cell infiltration, and metabolic conditions Full size image In summary, we have elucidated the distinct clonal architecture of EGFR mutation positive LUAD, providing insights as to how these may relate to the diverse clinical trajectories observed. While dominant truncal drivers, such as EGFR mutations are an important prerequisite for efficacious targeted therapies, the evolutionary trajectory for each tumor can be augmented by additional genomic events in the natural life history, enhancing clonal fitness with emergent drug resistance. Finally, we suggest that co-occurring truncal drivers and extent of genomic instability can have potential clinical value as biomarkers for risk stratification. Comprehensive depiction of the genomic landscape of EGFR -mutant LUAD may offer opportunities for development of high-precision therapeutic strategies tailored to individual risk of disease progression. Patient cohort and sample processing Among the patients diagnosed with LUAD at the National Cancer Centre Singapore, which underwent surgical resection of their tumors prior to receiving any form of therapy, 16 patients carrying EGFR mutations were selected for this study (relevant clinical information of each patient is provided in Supplementary Table 1 ). Written informed consent was obtained from all participating patients. The study was approved by the relevant Institutional Review Board (Singhealth Centralised IRB, Singapore). Resected tumors were sectioned horizontally and tumor tissue in each section was cut into four quadrants (A–D; Supplementary Fig. 1 ), which if large enough were processed further into smaller sectors. Pathologists’ evaluated sectors for reasonably high-tumor content were snap frozen for DNA/RNA sequencing. Neighboring horizontal sections were used for histological analyses. Adjacent normal lung tissue or blood was used as a matched normal control. DNA and total RNA extractions were performed from frozen tissues using Qiagen All prep universal kit and the DNA was subjected to library preparations for sequencing as described below. Whole-exome sequencing Quantity of 500 ng to 1 µg of genomic DNA was sheared using Covaris to a size of 300–400 bp and subjected to library preparation using NEBnext End repair, A-tailing and Ligation modules (New England Biolabs). 3–6 samples were pooled together and hybridized using the SeqCap EZ Human Exome Library v3.0 (Nimblegen, Roche) kit. Captured regions were washed, purified, amplified, and subjected to 2 × 101 sequencing on the Hiseq 2000 to obtain a mean coverage of 114X. Targeted amplicon deep sequencing Primers were designed around the somatic variants (SNVs and Indels) annotated to be in the exonic and splice regions, using the Generead DNA-seq custom panel v2 (Qiagen). In addition, primers covering the T790M locus in EGFR were also added to the panel. Amplicons were generated according to manufacturer’s recommendation and libraries were prepared using the NEBnext Ultra DNA-seq kit (New England Biolabs). Libraries were then pooled and sequenced on Hiseq 2500 by 150 bp paired end reads to obtain a mean depth of 3860X. SNV and indel calling from exome-seq Reads were mapped to the human reference sequence GRCh37 (hg19) using the bwa-aln algorithm [53] using default parameters. Duplicate reads were marked using Picard tools after which realignment around known indels and base quality recalibration was performed at an individual sample level using GATK 2.7 version [54] . Somatic mutation calling was performed using MuTect [55] allowing up to 5 reads supporting the variant allele in the normal sample up to a maximum of 0.05 allele frequency. The passed variants were further filtered using the described criteria to obtain a more confident set of somatic variants. A minimum of 6 reads supporting variant allele in the tumor was mandatory. To improve accuracy in low-frequency calls, variants with allele frequency (VAF) in tumor below 0.2 were treated as somatic only if the tumor allele frequency was at least 10 times greater than normal allele frequency for the variant allele. To eliminate false positive variant calls due to polymerase chain reaction (PCR)-chimeras formed in exome-seq protocols, germline variants were called from the normal sample of all patients as described below and were filtered out from the somatic variant list. Somatic indels were called using Strelka [56] and were further filtered for >4 reads (MAPQ >20) supporting the indel with a minimum allele frequency of 0.1. The final list of somatic SNVs and indels was then annotated by multiple databases using the Annovar tool [57] . Germline variant calling from exome-seq Germline variants for each patient were called from the normal sample using GATK Unified Genotyper after indel realignment and recalibration of bam files [54] . Variants were then subjected to hard filtering using GATK recommendations to obtain a more confident set of SNVs and indels. Variant calling from targeted deep-seq Fastq files were mapped to the human reference sequence GRCh37 (hg19) using bwa-mem algorithm with default parameters. The bam files were realigned and recalibrated using GATK. Since the amplicon size is around 150–200 bp, the reads obtained were overlapping. For each base at the overlapping region, if the pair bases were identical, quality score for both bases were updated to original quality score ×1.2; else if the pair bases were not identical, the base with the lower quality score was replaced by the base with the higher quality score, and both quality scores were updated to original higher quality scores ×0.8. Somatic SNVs were then called using VarScan v2.3.7 [58] . Default parameters were used except the minimum variant frequency was set to 0.01. Only those variants also called in the exome-seq were considered. Variants with <10 reads supporting the alternate allele were filtered out and variants with allele frequency below 0.05 were mandated to have a minimum alternate read count of 15. Further, mutation calls were required to have a VAF five times higher in the tumor compared to the normal. For somatic indels, read counts supporting the indel identified by exome-seq for that patient were obtained from both the tumor and normal bam files using a custom script. Reads properly paired and mapped with MAPQ >20 were counted. Somatic indels with >90% read counts from one strand were removed from further analyses. Further only those indels were treated as validated which had at least 10 reads supporting the alternate allele at a frequency five times greater in tumor than in normal with a minimum VAF of 0.03 in the tumor. A validation rate of 94% for indels and 85% for SNVs was achieved for the exome-seq data. Only validated variants were considered for generation of phylogenetic trees and any downstream analysis. Phylogenetic analysis Using the presence and absence of somatic mutations across samples, we first calculated the genetic distances between samples using the hamming distance. The neighbor joining algorithm from the APE package [59] was used to infer phylogenetic relationships between tumor sectors for each patient. Comparison with published data The published LUAD data sets [19] , [20] were retrieved from European Genome-phenome Archive (EGA). The corresponding EGA data set-IDs are: EGAS00001000930 and EGAD00001000900. In order to directly compare the pattern with our data set, we selected only those patients, where the tumor was restricted to a single site and had pure adenocarcinoma histology. The downloaded targeted deep sequencing data were processed using the same pipeline as our Singapore cohort data. Since the fraction of trunk mutations in the phylogenetic trees is a function of the number of sectors, we calibrated the trunk ratio by performing random subsampling of sectors for each patient. The average proportion of the trunk was compared across cases conditioning on the same number of sectors. Mutation signatures analysis In order to uncover mutational processes active within the EGFR mutant LUAD patients, we combined somatic mutations from the Singapore cohort with two published large-scale data sets [3] , [4] . With the information from the point mutation and the flanking 5′ and 3′ bases, the Emu package [60] was used to infer the mutation signatures in the 79 tumor sectors. Driver genes annotation We defined LUAD driver genes ( n = 78) through significantly mutated genes in LUAD collected from seven publications [1] , [2] , [3] , [4] , [61] , [62] , [63] . Mutations in these genes are shown to occur more than just by chance or due to the size of gene. Other cancer driver genes include additional significantly mutated genes in at least one cancer type from two pan cancer studies [62] , [63] and remaining genes in cancer gene census [64] ( n = 735). Non-silent mutations in these two lists of driver genes were annotated on the trees. For comparison across data sets, either LUAD genes or combined set of both groups of drivers (extended driver list) was used as indicated in main text or figure legends. Copy number analysis Illumina omniexpress arrays were run using DNA from all 79 tumor sectors along with matched normal tissue using protocols suggested by the manufacturer. Log ratio (LRR) and B allele frequency (BAF) for all SNPs on the array were obtained from Genome Studio. These LRR and BAF values were used as input for ASCAT [65] v2.4.1 along with the gender information. GC correction, followed by segmentation and purity/ploidy predictions along with obtaining allele-specific integer copy numbers was performed using ASCAT [65] . Each solution was manually checked and samples for which ASCAT could not provide a reliable solution (e.g., purity = 1) were eliminated from further analysis. 61 out of 79 samples from 15 patients remained after these filtering. For 5 of these 61 samples (namely A001-T-S03, A017-T-S10, A021-T-S02, A112-T-S28, and A112-T-S40), ASCAT solution was manually picked using second or third most optimal purity/ploidy solution since either the raw data suggested these sectors to be similar to other sectors from same patient or variant allele frequencies suggested alternate purity solution. While presence of multiple clones within a sector might lead to such alternate solutions in some scenarios [18] , [65] , we chose to be conservative in absence of a gold standard and removed any potentially artificial heterogeneity. Copy number losses or gains were determined relative to the median integer ploidy of the tumor which was obtained as the median integer copy number of the SNPs used in ASCAT analysis. Genomic Instability Index (GII) was calculated as the fraction of the total genome which was altered by any copy number gains or losses with copy change ≥1 defined relative to median integer ploidy. adGII (amplification and deletion based genomic instability index) scores were calculated as fraction of genome affected by high-copy gains and losses (or amplification and deletions with copy change ≥2 relative to ploidy). To obtain cytoband or gene level copy numbers, chromosomal locations of cytobands and genes were overlapped with those of the segments and the segment copy number was assigned to that cytoband or gene. In case multiple segments overlapped with the cytoband/gene, a minimum of 25% overlap was made mandatory and the segment with the highest overlap was used to assign the copy number to the cytoband/gene. Known driver regions in LUAD from previous large scale studies [4] , [6] , [7] , [8] , [41] were curated and only those regions were considered which were altered in same direction in at least two studies. Genome doubling status The genome doubling status for each tumor sample was determined using a published algorithm [38] . In brief, a p -value was obtained using 10,000 simulations with observed probabilities of copy number events. For samples with ploidy ≤3, a p -value threshold of 0.001 was used. To avoid underestimating genome doubling in high-ploidy samples, a p -value threshold of 0.05 was used for samples with ploidy = 4, and all samples were classified as genome doubled if the ploidy exceeds 4. Timing of mutations relative to copy number or genome doubling The cancer cell fraction (CCF) and mutant allele copy number for a given SNV was calculated following the algorithm described previously [16] , where the corresponding integer copy number and tumor purity were derived using SNP-array and ASCAT algorithm. A given mutation was classified as “clonal” if the 95% confidence interval of CCF overlapped 1, and “subclonal” otherwise. The timing of a given mutation relative to copy number alteration was classified on its clonal status and the integer rounded mutant allele copy number. Indels, regions with no copy number alteration (major copy number = minor copy number = 1), regions with just single copy were eliminated as these could not be evaluated for timing. Mutations were called early only when (i) the mutation is clonal, and (ii) the rounded integer mutant allele copy number ≥2. Dominance of the driver genes The dominance of a driver (driver self-sufficiency) was calculated for all known LUAD drivers ( n = 69) and ccRCC drivers ( n = 16) which were found mutated in ≥5 patients in the TCGA data. This was based on the logic that, for each cancer patient, the number of driver mutations found in each case implies the self-sufficiency of the drivers. Mutations which possess high capability to drive tumorigenesis would exist with few co-occurring driver mutations since these will be the sufficient to initiate a tumor. Using the combined public data sets [3] , [4] , we computed a measure for driver dominance of each gene as 
    D_ i = ∑_j = 1^N_ i 1/d_j/N_ i,
 where D i is the dominance score for gene i , N i is the number of patients carrying non-silent mutations in gene i while d j is the number of LUAD driver mutations in patient j . Therefore, the genetic dominance (i.e., self-sufficiency) ( D i ) we define is inversely proportional to the number of co-occurring driver mutations across samples. ccRCC drivers were picked from the TCGA publication as significantly mutated genes [42] . Cell culture 471L cells were derived from second generation of xenograft from A014 tumor (cells from first xenograft were transplanted into a second mouse). The tumor was collected, digested with 1 mg/ml Collagenase IV (Gibco, Life Technologies) and cultured on 100 mm plastic dish with culture conditions similar to those described earlier for patient-derived cell lines [24] . Using targeted sequencing we had confirmed that mutation found in the cell lines matched with the primary patient tumor (Supplementary Data 8 ). PC9-GefR cell line was generated by exposing PC9 cells (a gift from Dr. Sin Tiong Ong, Duke-NUS University, Singapore) to stepwise increment doses of Gefitinib (0.1–6.4 µM). Both isogenic cells were maintained in RPMI (Sigma-Aldrich), supplemented with 10% FBS (Hyclone, Fisher Scientific), 100 units/ml of Penicillin, 100 µg/ml of Streptomycin, and 0.25 µg/ml of Amphotericin B (Antibiotic-Antimycotic Gibco, Thermo Fisher Scientific). All cell lines were cultured in clean, well established cell culture labs with no sort of mycoplasma or other contamination. Dose response to Gefitinib 471L, PC9 and PC9-GefR cells were seeded into 96-well plates and were treated with varying concentration of drugs the next day (0.0001–20 µM). CellTiter-Glo Reagent (Promega) was added directly to the cells per manufacturer’s instructions after a 72 h treatment period. Luminescence was measured to determine the amount of viable cells. Percentage cell viability was calculated relative to 0.2% DMSO vehicle control. All cell viability assays were performed in triplicates. Dose response curves were generated using GraphPad Prism version 7. Data availability All the sequencing and SNP array data have been deposited at the European Genome-phenome Archive (EGA, http://www.ebi.ac.uk/ega/ ), which is hosted by the EBI, under the accession code EGAS00001001736.